Epigenetic regulation of Smad2 and Smad3 by profilin-2 promotes lung cancer growth and metastasis Altered transforming growth factor-β (TGF-β) signalling has been implicated in tumour development and progression. However, the molecular mechanism behind this alteration is poorly understood. Here we show that profilin-2 (Pfn2) increases Smad2 and Smad3 expression via an epigenetic mechanism, and that profilin-2 and Smad expression correlate with an unfavourable prognosis of lung cancer patients. Profilin-2 overexpression promotes, whereas profilin-2 knockdown drastically reduces, lung cancer growth and metastasis. We show that profilin-2 suppresses the recruitment of HDAC1 to Smad2 and Smad3 promoters by preventing nuclear translocation of HDAC1 through protein–protein interaction at the C terminus of both proteins, leading to the transcriptional activation of Smad2 and Smad3. Increased Smad2 and Smad3 expression enhances TGF-β1-induced EMT and production of the angiogenic factors VEGF and CTGF. These findings reveal a new regulatory mechanism of TGF-β1/Smad signalling, and suggest a potential molecular target for the development of anticancer drugs. Cancer is a major threat for health worldwide. Despite tremendous advancements in combating human cancers, the mechanism underlying the occurrence and progression of many types of cancers remains to be further characterized. Transforming growth factor-β (TGF-β) is a signal molecule with multiple cellular functions. It plays important roles in regulating embryogenesis, tissue homeostasis and various pathophysiological events. TGF-β has been shown to be a critical regulator of tumorigenesis and tumour metastasis. Alteration of TGF-β signalling has been linked to the progression of cancers [1] . Previous reports have demonstrated that TGF-β signalling and the subsequent biological events such as the epithelial-to-mesenchymal transition (EMT) and angiogenesis are involved in the growth, invasion and metastasis of cancers [2] , [3] , [4] , [5] , [6] , [7] . Due to the critical function of TGF-β as a pro-tumour factor, there has been increasing interests in targeting the TGF-β pathway for cancer interventions [8] . Changes of TGF-β signalling components during cancer development and progression have been observed in various primary and metastatic tumours [9] . It is important to further deepen our understanding of the regulation of TGF-β signalling in cancer progression. Current investigations on regulation of TGF-β signalling are primarily focused on ubiquitination- and sumoylation-related events. It has been reported that various ubiquitin ligases play important roles in the degradation of TGF-β receptors and Smads through the ubiquitin–proteasome pathway. By contrast, the SUMO ligases are responsible for stabilising TGF-β receptors and Smads [10] , [11] . Profilins (pro-filamentous actins, Pfns) are well-known actin-binding proteins [12] . Profilin-1 (Pfn1) and profilin-2 (Pfn2) are the most abundant profilins in mammalian cells. These two profilin variants have similar actin monomer-binding properties [13] . In the presence of formin, profilin promotes the elongation of the uncapped barbed end of the actin filament. When the barbed ends are capped, profilin promotes the disassembly of the actin filament [14] . Although profilin-1 and profilin-2 have similar properties, only profilin-1 is an essential molecule that shows dose-dependent effects on cell division and survival during embryogenesis in mice. The loss of proflin-1 cannot be compensated by profilin-2 (ref. 15 ). Mice lacking profilin-2 display blocked synaptic actin polymerization in response to depolarization, accompanied by increased synaptic excitability in glutamatergic neurons due to the increased vesicle exocytosis [16] . It has also been reported that profilin-1 regulates blastopore closure. Manipulation of profilin-1expression specifically affects convergent extension movement. Profilin-2 modulates the cell polarization and axial alignment of mesodermal cells at gastrulation stage in a profilin-1-independent manner [17] , [18] . These observations suggest that profilin-1 and profilin-2 may play non-redundant roles in early embryonic development. Profilin-1 has been reported to be involved in the control of breast cancer progression. Profilin-1 can function as a negative regulator for the growth and migration of breast cancer cells [19] , [20] , [21] , [22] , [23] . However, a recent report has suggested the opposite roles of profilin-1 and profilin-2 in the migration and invasion of breast cancer cells [24] . Another recent report suggested that profilin-1 played dual roles at different stages of breast cancer progression [25] . Thus, the role of profilin in cancer progression and the mechanism of it remain to be further clarified. In this study, we investigated the roles of profilin-2 in human lung cancer progression and its link with the TGF-β/Smad signalling. We show that profilin-2 suppresses the nuclear localization of histone deacetylase 1 (HDAC1) by interacting with HDAC1, which epigenetically activates the transcription of Smad2 and Smad3 and thereby promotes human lung cancer growth and metastasis. Our study provides an insight into how TGF-β/Smad signalling is regulated in lung cancers, and suggests a new molecular target for drug development. Correlation between profilin and Smad3 in human lung cancers By analysing the expression profiles of profilin and Smad3 in different GEO data sets (accession codes GSE1643, GSE4127 and GSE4573), we found a potential regulatory effect of profilin-2 on Smad levels in cancer progression. Compared with normal lung tissues, profilin-2 messenger RNA (mRNA) levels were significantly upregulated in human lung cancer cell lines and lung cancer tissues ( Fig. 1a ). The expressions levels of profilin-2 and Smad3 were positively correlated in human lung cancer cell lines ( Fig. 1b ) and human lung cancer tissues ( Fig. 1c ). The slope values of the regression lines (0.775 in lung cancer cell lines and 2.2925 in lung cancer tissues) indicated that the expression levels of profilin-2 and Smad3 were highly correlated ( Fig. 1b,c ). By comparing the profilin-2 H-scores in cancer tissues and the adjacent tissues from 106 lung cancer patients, we found that the profilin-2 protein levels were significantly increased in cancer tissues compared with the adjacent tissues in 88.68% of patients. No obvious change of profilin-2 protein levels was detected in 10.38% of the patients, and only 0.95% of the patients showed decreased profilin-2 expression level in cancer tissues ( Fig. 1d ). These data suggest that profilin-2 expression was significantly increased in lung cancer tissues. Furthermore, high profilin-2 level (H-score≥5) in cancer tissues was linked to poor survival rate in lung cancer patients ( Fig. 1e ). By analysing the profilin-2 and Smad3 levels in 106 lung cancer samples, we observed a positive correlation between profilin-2 and Smad3 mRNA levels ( R =0.9411, a =0.4903; Fig. 1f ). A similar positive correlation between the profilin-2 and Smad3 protein levels in several human lung cancer cell lines was also observed ( Fig. 1g ). The profilin-1 mRNA level decreased significantly in lung cancer cell lines and tissues ( Fig. 1h ), but no statistically significant correlations between profilin-1 and Smad3 expressions was observed ( Fig. 1i,j ). These data suggest that profilin-2 may function as a potential activator of Smad3 expression in human lung cancer cells. Increased Smad3 expression level may be important for the development and progression of cancers. 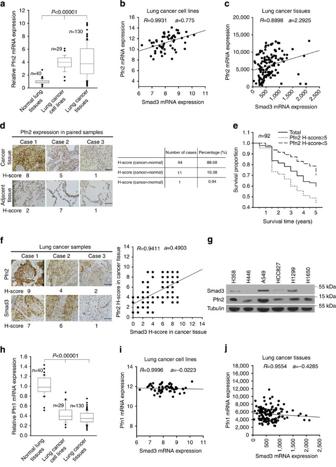Figure 1: The correlation between the expression levels of Pfn2 and Smad3 in human lung cancer. (a) Pfn2 mRNA is upregulated in human lung cancer cell lines and cancer tissues. The data are from GEO data sets GSE1643, GSE4127 and GSE4573. ANOVA test,P<0.00001, error bars represent the means±s.e.m. of indicated samples. (b,c) The relationship between the levels of Smad3 and Pfn2 in various lung cancer cells and lung cancer tissues. (d) The representative (left) and statistic (right) results of immunohistochemistry staining of Pfn2 in paired human normal lung and cancer tissues. Scale bar, 200 μm. (e) The relationship between the Pfn2 expression and lung cancer patient survival rate. (f) The representative (left) results of immunohistochemistry staining of Pfn2 and Smad3 in human lung cancer samples. The relationship between Pfn2 and Smad3 protein levels was also shown in the right panel. Scale bar, 200 μm. (g) Pfn2 and Smad3 protein expressions in human lung cancer cell lines were detected by western blotting. One representative result of three experiments is shown. (h) Pfn1 mRNA is decreased in human lung cancer cell lines and tissues. The data are from GEO data sets GSE1643, GSE4127 and GSE4573. ANOVA test,P<0.00001, error bars represent the means±s.e.m. of indicated samples. (i,j) The relationship between the levels of Smad3 and Pfn1 in various lung cancer cells and lung cancer tissues. The data are from GEO data sets GSE1643, GSE4127 and GSE4573. ANOVA, analysis of variance. Figure 1: The correlation between the expression levels of Pfn2 and Smad3 in human lung cancer. ( a ) Pfn2 mRNA is upregulated in human lung cancer cell lines and cancer tissues. The data are from GEO data sets GSE1643, GSE4127 and GSE4573. ANOVA test, P <0.00001, error bars represent the means±s.e.m. of indicated samples. ( b , c ) The relationship between the levels of Smad3 and Pfn2 in various lung cancer cells and lung cancer tissues. ( d ) The representative (left) and statistic (right) results of immunohistochemistry staining of Pfn2 in paired human normal lung and cancer tissues. Scale bar, 200 μm. ( e ) The relationship between the Pfn2 expression and lung cancer patient survival rate. ( f ) The representative (left) results of immunohistochemistry staining of Pfn2 and Smad3 in human lung cancer samples. The relationship between Pfn2 and Smad3 protein levels was also shown in the right panel. Scale bar, 200 μm. ( g ) Pfn2 and Smad3 protein expressions in human lung cancer cell lines were detected by western blotting. One representative result of three experiments is shown. ( h ) Pfn1 mRNA is decreased in human lung cancer cell lines and tissues. The data are from GEO data sets GSE1643, GSE4127 and GSE4573. ANOVA test, P <0.00001, error bars represent the means±s.e.m. of indicated samples. ( i , j ) The relationship between the levels of Smad3 and Pfn1 in various lung cancer cells and lung cancer tissues. The data are from GEO data sets GSE1643, GSE4127 and GSE4573. ANOVA, analysis of variance. Full size image Profilins play different roles in lung tumour progression To determine the roles of profilin in lung tumour growth and metastasis, we overexpressed or knocked down profilin-1 and profilin-2 in A549 cells ( Fig. 2a ). The cells were subcutaneously injected into nude mice. Profilin-2 overexpression strongly promoted lung tumour growth, and its knockdown suppressed tumour growth. However, neither profilin-1 overexpression nor its knockdown showed obvious effect on tumour growth ( Fig. 2b,c ). No significant effect of profilin overexpression or knockdown on A549 cell proliferation was observed ( Supplementary Fig. 1a,b ). Consistently, no obvious effect of profilin on the cell cycle was detected ( Supplementary Fig. 1c ). In addition, neither profilin-1 overexpression nor its knockdown showed obvious effect on the ability of colony formation in soft agar ( Supplementary Fig. 1d ). However, profilin-2 overexpression and knockdown significantly increased and suppressed, respectively, the colony formation of lung cancer cells ( Supplementary Fig. 1d,e ). These results suggest that the increased anchorage-independent cell growth mediated by profilin-2 may contribute to enhanced lung tumour growth. The circulating tumour cell (CTC) concentration was also dependent on the expression level of profilin-2. Overexpression of profilin-1 did not affect the relative CTC concentration, whereas knockdown of profilin-1 significantly increased the relative CTC concentration ( Fig. 2d ). We also analysed the invasiveness of cancer cells by in vitro matrigel invasion assay. Overexpression of profilin-2 significantly increased the matrigel invasion ability of lung cancer cells. Knocking down profilin-2 had the opposite effect on the lung cancer cell invasion ability to overexpression. Overexpression of profilin-1 did not affect the lung cancer cell invasive ability, whereas knocking down profilin-1 significantly increased the matrigel invasion of lung cancer cells ( Supplementary Fig. 1f,g ). These results suggest that profilin-2 is a potent factor to enhance lung tumour growth. Although profilin-1 did not affect lung tumour growth, low profilin-1 expression facilitated lung tumour invasion, suggesting that profilin-1 is involved in modulating the metastasis of lung cancer cells. 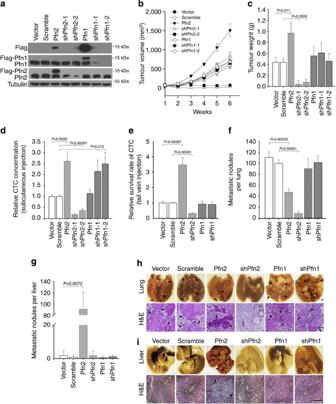Figure 2: The effects of profilins on lung cancer growth, invasion and metastasis. (a) The stable Pfns-overexpressing or knockdown A549 cell lines were prepared using a lentiviral system. Western blotting result of three experiments is shown. (b,c) Effects of Pfns on lung cancer growth as determined by tumour volume and tumour weight. Student’st-test is used for statistical analysis of vector versus Pfn2, ANOVA test for statistic comparison of vector, shPfn2-1 and shPfn2-2; thePvalues are shown in the figure. (d) The relative circulating tumour cell (CTC) concentration was detected 6 weeks after tumour transplantation. Student’st-test is used for statistical analysis of vector versus Pfn2, and ANOVA test for comparison of other groups, thePvalues are shown in the figure. (e) The relative CTC concentration was detected 2 months after tail-vein injection. Student’st-test is used for statistical analysis, thePvalues are shown in the figure. (f–i) The effect of Pfn on lung and liver metastasis was determined by the number of metastatic nodules, morphology and H&E staining. Arrows indicate exemplary loci of metastasis. Scale bar, 200 μm. All error bars in the figure represent the means±s.d. of three independent experiments (five mice per group for all groups). ANOVA, analysis of variance; H&E, haematoxylin and eosin. Figure 2: The effects of profilins on lung cancer growth, invasion and metastasis. ( a ) The stable Pfns-overexpressing or knockdown A549 cell lines were prepared using a lentiviral system. Western blotting result of three experiments is shown. ( b , c ) Effects of Pfns on lung cancer growth as determined by tumour volume and tumour weight. Student’s t -test is used for statistical analysis of vector versus Pfn2, ANOVA test for statistic comparison of vector, shPfn2-1 and shPfn2-2; the P values are shown in the figure. ( d ) The relative circulating tumour cell (CTC) concentration was detected 6 weeks after tumour transplantation. Student’s t -test is used for statistical analysis of vector versus Pfn2, and ANOVA test for comparison of other groups, the P values are shown in the figure. ( e ) The relative CTC concentration was detected 2 months after tail-vein injection. Student’s t -test is used for statistical analysis, the P values are shown in the figure. ( f – i ) The effect of Pfn on lung and liver metastasis was determined by the number of metastatic nodules, morphology and H&E staining. Arrows indicate exemplary loci of metastasis. Scale bar, 200 μm. All error bars in the figure represent the means±s.d. of three independent experiments (five mice per group for all groups). ANOVA, analysis of variance; H&E, haematoxylin and eosin. Full size image The survival of CTC is one of the most important factors influencing the formation of distal metastasis; we analysed the survival rate of CTC by determining the relative CTC concentration after tail-vein injection of A549 lung cancer cells. Profilin-2 overexpression significantly increased the survival rates of CTC, whereas profilin-2 knockdown strongly decreased the survival rates of CTC ( Fig. 2e ). In addition, profilin-2 overexpression decreased lung metastatic nodules and markedly promoted liver metastasis, whereas its knockdown almost abolished the lung and liver metastasis ( Fig. 2f–i ). These results demonstrated that profilin-2 is essential for lung tumour growth and liver metastasis. The results that profilin-2 overexpression increased the survival of CTC while decreased lung metastasis also suggest that profilin-2 negatively impacted the extravasation ability of lung cancer cells in lung. Unlike profilin-2, variation of profilin-1 expression did not affect the survival rate of CTC in the blood ( Fig. 2e ). Consistently, profilin-1 did not affect the metastatic formation of lung tumour either ( Fig. 2f–i ). These observations suggest that profilin-2 can enhance lung cancer growth and liver metastasis, while profilin-1 functions as a suppressor of the invasion and vascular dissemination of lung cancers. Further investigation showed that overexpression of mouse Pfn2 (mPfn2) rescued the in vitro soft agar colony formation and matrigel invasion abilities of profilin-2 knockdown cells ( Supplementary Fig. 2a–c ). The suppressive effects of profilin-2 knockdown on lung tumour growth, CTC concentration, liver and lung metastasis were also rescued by overexpression of mPfn2 ( Supplementary Fig. 2d–h ). The role of Pfn2 in liver colonization of lung cancer cells In addition to the ability to invade and survive in the circulating blood, tumour cells require other factors to facilitate the organ metastasis. The ‘seeding’ or the colonization step determines whether the tumour cells in blood are able to settle down in distal organs or tissues. Profilin-2 is likely to be one of the determining factors at the seeding step during the metastatic journey of lung cancer cells. We performed experiments to test this hypothesis. The profilin-2-overexpressing or knockdown A549 cells were added to dishes with confluent primary hepatocytes. Seven days later, puromycin was added to kill the primary hepatocytes to visualize the colonies formed by puromycin-resistant A549 cells. Profilin-2 overexpression induced the formation of lung cancer cell colonies in dishes coated with primary hepatocytes ( Supplementary Fig. 3a ). When primary hepatocytes were co-cultured with profilin-2-overexpressing lung cancer cells pre-seeded in dishes, no increased colony formation was observed, indicating that profilin-2 overexpression did not provide the lung cancer cells with a growth advantage in an environment surrounded by primary hepatocytes ( Supplementary Fig. 3b ). These results suggest that profilin-2 promotes liver metastasis by increasing liver seeding of lung cancer cells. Because profilins are important regulators of F-actin dynamics, there is a possibility that profilin-2 regulates tumour growth and metastasis by modulating the F-actin dynamics. However, we found that neither overexpression nor knockdown of profilin-2 had any significant effects on the morphology and F-actin pattern of A549 cells ( Supplementary Fig. 4a,b ). Although these results cannot rule out the actin-dependent function of profilin-2 in lung cancer progression, they suggest a possibility that other unknown mechanism can be involved in profilin-2-mediated lung cancer progression. Profilin-2 activates the TGF-β/Smad signalling pathway Because the profilin-2 and Smad3 levels are closely correlated, we investigated whether profilin-2 functions through the TGF-β/Smad signalling pathway. TGF-β activities in profilin overexpression and profilin knockdown cells were detected using (CAGA) 12 and (SBE) 4 luciferase TGF-β reporter systems. Profilin-2 overexpression significantly increased the TGF-β signalling, and profilin-2 knockdown decreased the TGF-β signalling. The TGF-β signalling was not affected by either the overexpression or knockdown of profilin-1 ( Fig. 3a ). Moreover, profilin-2 overexpression increased Smad2 and/or Smad3 protein expression levels in A549, HCC827 and H1650 cells, whereas profilin-2 knockdown decreased Smad2 and Smad3 protein expression levels in A549 and H1650 cells. Neither the overexpression nor knockdown of profilin-2 affected the expression of Smad4 ( Fig. 3b ). Further investigation showed that profilin-2 overexpression and knockdown increased and reduced, respectively, the Smad2 and Smad3 nuclear translocation in lung cancer cells ( Fig. 3c ; Supplementary Table 1 ). Profilin-2 overexpression also enhanced TGF-β1-mediated Smad2 and Smad3 phosphorylation, while its knockdown attenuated the phosphorylation in A549 cells ( Fig. 3d ). These results suggest that profilin-2 is a potent activator of Smad2 and Smad3 expression. 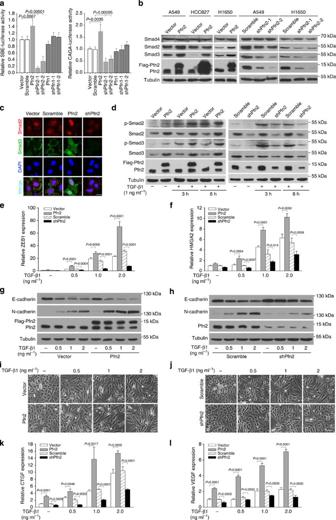Figure 3: Pfn2 is an activator of TGF-β/Smad signalling pathway. (a) The effects of Pfns overexpression and knockdown on (CAGA)12and (SBE)4luciferase activities of TGF-β reporter systems. Student’st-test is used for comparison of vector versus Pfn2, and ANOVA test for comparison of scramble, shPfn2-1 and shPfn2-2. ThePvalues are shown in the figure. (b) Western blotting analysis of Smad expression in Pfn2 overexpression and knockdown cells. One representative result of three independent experiments is shown. (c) Co-immunofluorescent staining of Smad2 and Smad3 in indicated cells. Red colour represents Smad2, green colour represents Smad3 and the blue colour represents the nucleus. Scale bar, 20 μm. (d) The effects of overexpression (right) and knockdown (left) of Pfn2 on TGF-β1-mediated Smad2 and Smad3 phosphorylation in A549 cells. One representative western blotting result of three experiments was shown. (e,f) mRNA levels of ZEB1 and HMGA2 were detected by real-time PCR. Student’st-test, thePvalues are shown in the figure. (g,h) EMT marker proteins E-cadherin and N-cadherin were examined after treatment with indicated concentration of TGF-β1 for 2 days. One representative western blotting result of three experiments is shown. (i,j) The morphology changes of indicated cell lines were photographed after treatment with indicated concentration of TGF-β1 for 2 days. Scale bar, 20 μm. (k,l) mRNA levels of CTGF and VEGF were detected by real-time PCR. Student’st-test is used for statistical analysis; thePvalues are shown in the figure. All error bars in the figure represent the means±s.d. of four independent experiments. ANOVA, analysis of variance. Figure 3: Pfn2 is an activator of TGF-β/Smad signalling pathway. ( a ) The effects of Pfns overexpression and knockdown on (CAGA) 12 and (SBE) 4 luciferase activities of TGF-β reporter systems. Student’s t -test is used for comparison of vector versus Pfn2, and ANOVA test for comparison of scramble, shPfn2-1 and shPfn2-2. The P values are shown in the figure. ( b ) Western blotting analysis of Smad expression in Pfn2 overexpression and knockdown cells. One representative result of three independent experiments is shown. ( c ) Co-immunofluorescent staining of Smad2 and Smad3 in indicated cells. Red colour represents Smad2, green colour represents Smad3 and the blue colour represents the nucleus. Scale bar, 20 μm. ( d ) The effects of overexpression (right) and knockdown (left) of Pfn2 on TGF-β1-mediated Smad2 and Smad3 phosphorylation in A549 cells. One representative western blotting result of three experiments was shown. ( e , f ) mRNA levels of ZEB1 and HMGA2 were detected by real-time PCR. Student’s t -test, the P values are shown in the figure. ( g , h ) EMT marker proteins E-cadherin and N-cadherin were examined after treatment with indicated concentration of TGF-β1 for 2 days. One representative western blotting result of three experiments is shown. ( i , j ) The morphology changes of indicated cell lines were photographed after treatment with indicated concentration of TGF-β1 for 2 days. Scale bar, 20 μm. ( k , l ) mRNA levels of CTGF and VEGF were detected by real-time PCR. Student’s t -test is used for statistical analysis; the P values are shown in the figure. All error bars in the figure represent the means±s.d. of four independent experiments. ANOVA, analysis of variance. Full size image Because TGF-β-induced EMT has been implicated in lung tumour cell migration and metastasis [26] , [27] , it is important to know whether the profilin-2–Smad pathway is linked to TGF-β-induced EMT. The overexpression of profilin-2 significantly enhanced the TGF-β1-induced expression of ZEB1, an EMT-inducing transcription factor. By contrast, the knockdown of profilin-2 significantly suppressed TGF-β1-induced ZEB1 expression ( Fig. 3e ). Similar results were also obtained by examining the expression levels of HMGA2 ( Fig. 3f ) and SNAI1/SNAI2 ( Supplementary Fig. 5a,b ). In addition, the TGF-β1-induced changes in the levels of E-cadherin and N-cadherin were enhanced by profilin-2 overexpression. In contrast, profilin-2 knockdown suppressed these effects of TGF-β1 ( Fig. 3g,h ; Supplementary Fig. 5c,d ). Moreover, the overexpression or knockdown of profilin-2 also significantly promoted or suppressed, respectively, the morphological changes induced by TGF-β1 in A549 cells ( Fig. 3i,j ). The above results indicate that profilin-2 activates TGF-β1-induced EMT in human lung cancer cells. Angiogenesis has been shown to be important for TGF-β-mediated cancer progression. Vascular endothelial growth factor (VEGF) and connective tissue growth factor (CTGF) are angiogenesis factors that can be regulated by TGF-β. Interestingly, profilin-2 overexpression or knockdown significantly upregulated or decreased, respectively, the expression of VEGF and CTGF. Profilin-2 overexpression or knockdown also significantly enhanced or suppressed, respectively, the TGF-β1-induced VEGF and CTGF expression ( Fig. 3k,l ). These results suggest that profilin-2 enhance the tumour growth and metastasis via a mechanism involving the activation of TGF-β1-induced EMT and the expression of angiogenic factors. Smad is essential for Pfn2-mediated lung cancer progression To determine whether Smad plays a role in profilin-2-mediated lung tumour growth and metastasis, we examined the effect of Smad knockdown. Notably, the knockdown of Smad2 and Smad3 in profilin-2-overexpressing cells suppressed lung tumour growth ( Fig. 4a–c ), decreased the relative CTC concentration ( Fig. 4d ), inhibited lung ( Fig. 4e,h ) and liver ( Fig. 4f,i ) metastatic nodule formation and reduced the survival rate of CTC in mice( Fig. 4g ). Smad2 and Smad3 knockdown had no obvious effect on the proliferation rate of lung cancer cells ( Fig. 4j ) but significantly suppressed the anchorage-independent growth stimulated by profilin-2 overexpression ( Fig. 4k ). Moreover, the profilin-2 overexpression stimulated in vitro matrigel invasion of lung cancer cells was markedly reduced ( Fig. 4l ). 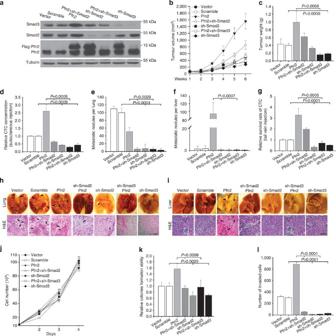Figure 4: Smad2 and Smad3 are essential for Pfn2-mediated effects. (a) The expressions of Smads were examined by western blotting. One representative result of three experiments is shown. (b–i) The effects of Smad2 and Smad3 knockdown in Pfn2-overexpressing cells on lung cancer growth, CTC concentration and metastasis: tumour volume, weight, CTC concentration, lung and liver metastasis, and survival rate in blood. Student’st-test is used for comparison of two groups and ANOVA test for comparison of more than two groups; thePvalues are shown in figure. Error bars represent the means±s.d. of three independent experiments (five mice per group for all groups). Scale bar, 200 μm. (j) Knockdown of Smad2 and Smad3 has no significant effects on the proliferation of A549 cells as determined by cell number counting. Error bars represent the means±s.d. of four independent experiments. (k) The statistical results of soft agar colonies formation assay. ANOVA test; thePvalues are shown in the figure. Error bars represent the means±s.d. of four independent experiments. (l) The statistical results of matrigel invasion assays. ANOVA test; thePvalues are shown in the figure. Error bars represent the means±s.d. of three independent experiments. ANOVA, analysis of variance. Figure 4: Smad2 and Smad3 are essential for Pfn2-mediated effects. ( a ) The expressions of Smads were examined by western blotting. One representative result of three experiments is shown. ( b – i ) The effects of Smad2 and Smad3 knockdown in Pfn2-overexpressing cells on lung cancer growth, CTC concentration and metastasis: tumour volume, weight, CTC concentration, lung and liver metastasis, and survival rate in blood. Student’s t -test is used for comparison of two groups and ANOVA test for comparison of more than two groups; the P values are shown in figure. Error bars represent the means±s.d. of three independent experiments (five mice per group for all groups). Scale bar, 200 μm. ( j ) Knockdown of Smad2 and Smad3 has no significant effects on the proliferation of A549 cells as determined by cell number counting. Error bars represent the means±s.d. of four independent experiments. ( k ) The statistical results of soft agar colonies formation assay. ANOVA test; the P values are shown in the figure. Error bars represent the means±s.d. of four independent experiments. ( l ) The statistical results of matrigel invasion assays. ANOVA test; the P values are shown in the figure. Error bars represent the means±s.d. of three independent experiments. ANOVA, analysis of variance. Full size image To further confirm the role of Smad2 and Smad3 in the function of profilin-2 in lung cancer growth and metastasis, we examined the effect of Smad overexpression on profilin-2 knockdown cells ( Supplementary Fig. 6a ). Smad2 and Smad3 overexpression significantly rescued the suppressive effect of profilin-2 knockdown on soft agar colony formation of lung cancer cells ( Supplementary Fig. 6b ). Smad2 and Smad3 overexpression also partially rescued the matrigel invasion ability of profilin-2 knockdown cells ( Supplementary Fig. 6c ). These results indicate that Smad2 and Smad3 are important in profilin-2-mediated lung cancer progression. Epigenetic regulation of Smad promoters by Pfn2 To investigate the mechanism of profilin-2 in regulating Smad signalling, we examined the effect of profilin-2 on Smad mRNA expression. Profilin-2 overexpression and knockdown significantly increased and decreased, respectively, the mRNA levels of Smad2 and Smad3 ( Fig. 5a ). Profilin-2 overexpression and knockdown also increased and decreased, respectively, the transcriptional activity of Smad2 and Smad3 promoters ( Fig. 5b ). These results indicate that profilin-2 activates Smad2 and Smad3 transcription. Profilin-2 is localized primarily in the cytoplasm, and its overexpression has no effect on its subcellular localization ( Fig. 5c,j,k ), implying that profilin-2 activates Smad2 and Smad3 transcription by an indirect way. Since epigenetic modification is an important mechanism in the control of various cellular functions, we examined whether profilin-2 regulates Smad2 and Smad3 expression through the epigenetic modification of their promoters. Profilin-2 overexpression significantly increased the histone acetylation levels at the transcriptional activation sites (H2AK5, H2BK12 and H3K9/14) [28] of Smad2 promoter, whereas its knockdown decreased the acetylation levels of H2BK12 ( Fig. 5d ). Profilin-2 overexpression increased the acetylation levels of H2AK5 and H2BK12 in Smad3 promoter, and its knockdown decreased the acetylation levels of H3K9/14 in Smad3 promoter ( Fig. 5e ). Because histone acetylation and methylation are two closely interacting processes [29] , [30] , [31] , we also detected the histone tri-methylation levels at the transcriptional inhibition sites (H3K9 and H3K27) [28] and a transcriptional activation site (H3K4) [32] , [33] , [34] of Smad promoters. Profilin-2 overexpression significantly decreased the tri-methylation levels of H3K9 and H3K27, and its knockdown significantly increased the tri-methylation levels of H3K27 of Smad2 promoter ( Fig. 5f ). The increased tri-methylation of H3K4 and decreased tri-methylation of H3K9 in Smad3 promoter were also induced by profilin-2 overexpression. Conversely, increased tri-methylation of H3K9 and H3K27 in Smad3 promoter was induced by profilin-2 knockdown ( Fig. 5g ). These results suggest that profilin-2 activates Smad2 and Smad3 expression by regulating the histone modifications of their promoters. 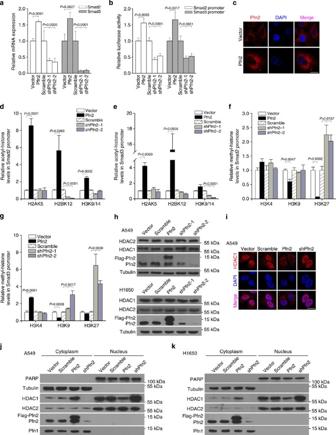Figure 5: Pfn2 regulates the epigenetic states of Smad promoters through HDAC1. (a) Smad2 and Smad3 mRNA expressions were examined by real-time PCR. (b) The luciferase activities of Smad2 and Smad3 promoters were determined using the Dual-Luciferase Reporter Assay System (see the Method section). (c) Immunofluorescent staining of Pfn2 in control and Pfn2-overexpressing cells. Red colour represents Pfn2 and blue colour represents nucleus. Scale bar, 20 μm. (d,e) Effects of Pfn2 on histone acetylation of H2AK5, H2BK12 and H3K9/14 at the promoters of Smad2 and Smad3. (f,g) Effects of Pfn2 on histone tri-methylation of H3K4, H3K9 and H3K27 at the promoters of Smad2 and Smad3. (h)The expression of HDAC1 and HDAC2 was detected by western blotting. One representative result of three experiments is shown. (i) Immunofluorescent staining of HDAC1 in indicated cells. Red colour represents HDAC1 and blue colour represents nucleus. Scale bar, 20 μm. (j,k) Cellular localization of HDACs in A549 and H1650 cells was detected by western blotting. One representative result of three experiments is shown. For the statistical analysis in this figure, Student’st-test is used for comparison of vector versus Pfn2; ANOVA test is used for comparison of scramble, shPfn2-1 and shPfn2-2. All thePvalues are shown in the figure. Error bars represent the means±s.d. of four independent experiments. ANOVA, analysis of variance; DAPI, 4′,6′-diamidino-2-phenylindole. Figure 5: Pfn2 regulates the epigenetic states of Smad promoters through HDAC1. ( a ) Smad2 and Smad3 mRNA expressions were examined by real-time PCR. ( b ) The luciferase activities of Smad2 and Smad3 promoters were determined using the Dual-Luciferase Reporter Assay System (see the Method section). ( c ) Immunofluorescent staining of Pfn2 in control and Pfn2-overexpressing cells. Red colour represents Pfn2 and blue colour represents nucleus. Scale bar, 20 μm. ( d , e ) Effects of Pfn2 on histone acetylation of H2AK5, H2BK12 and H3K9/14 at the promoters of Smad2 and Smad3. ( f , g ) Effects of Pfn2 on histone tri-methylation of H3K4, H3K9 and H3K27 at the promoters of Smad2 and Smad3. ( h )The expression of HDAC1 and HDAC2 was detected by western blotting. One representative result of three experiments is shown. ( i ) Immunofluorescent staining of HDAC1 in indicated cells. Red colour represents HDAC1 and blue colour represents nucleus. Scale bar, 20 μm. ( j , k ) Cellular localization of HDACs in A549 and H1650 cells was detected by western blotting. One representative result of three experiments is shown. For the statistical analysis in this figure, Student’s t -test is used for comparison of vector versus Pfn2; ANOVA test is used for comparison of scramble, shPfn2-1 and shPfn2-2. All the P values are shown in the figure. Error bars represent the means±s.d. of four independent experiments. ANOVA, analysis of variance; DAPI, 4′,6′-diamidino-2-phenylindole. Full size image To understand how profilin-2 regulates the histone modification levels of Smad promoters, we also investigated the effect of profilin-2 on the HDAC expression and subcellular localization. Although profilin-2 overexpression and knockdown had no obvious effect on the expression levels of HDAC1 and HDAC2 ( Fig. 5h ), its overexpression or knockdown significantly decreased or increased, respectively, the nuclear localization of HDAC1 in different human lung cancer cell lines ( Fig. 5i–k ; Supplementary Table 1 ). Profilin-2 has no obvious effect on the cellular localization of HDAC2 ( Fig. 5j,k ). In addition, neither the overexpression nor knockdown of profilin-1 affected the expression and cellular localization of HDAC1 and HDAC2 ( Supplementary Fig. 7a–d ). These results suggest that profilin-2 inhibits the nuclear translocation of HDAC1 to release its inhibition of Smad2 and Smad3 expression. The Pfn2–HDAC1 interaction is important for Smad expression To investigate how profilin-2 reduces the nuclear location of HDAC1, we examined whether there is any interaction between profilin-2 and HDAC1. Immunoprecipitation assay showed that profilin-2 can bind with HDAC1 but not HDAC2 ( Fig. 6a ). Immunoprecipitation assay using flag-tagged profilin-2 and myc-tagged HDAC2 confirmed that profilin-2 does not interact with HDAC2 ( Supplementary Fig. 8 ). In addition, neither HDAC1 nor HDAC2 can bind profilin-1 ( Fig. 6a ). These results suggest that profilin-2 sequestrates HDAC1 in the cytoplasm through protein–protein interaction. In mammalian cells, alternative splicing can occur at the C terminus of profilin-2, which results in two splicing variants (profilin-2a and profilin-2b). Because profilin-2b is a rare variant, the profilin-2 used in our investigation is profilin-2a. The alternative splicing C terminus of profilin-2 is relatively conserved and may be responsible for its distinct biological functions [13] , [35] . Thus, we next examined whether the C terminus of profilin-2 is essential for its binding with HDAC1. We constructed an N-residue deletion profilin-2 plasmid (ΔN-Pfn2, amino acids 29–140) and a C-residue deletion profilin-2 plasmid (ΔC-Pfn2, amino acids 1–108; ( Fig. 6b , upper panel), and detected their HDAC1-binding abilities. The full-length Pfn2 and the ΔN-Pfn2, but not theΔC-Pfn2, interacted with HDAC1 ( Fig. 6c ). Moreover, the overexpression of full-length Pfn2 and ΔN-Pfn2 increased the mRNA and protein expression of Smad2 and Smad3 ( Fig. 6d ; Supplementary Fig. 9 ) and inhibited the nuclear location of HDAC1 ( Fig. 6e ). These effects could not be generated by the overexpression of ΔC-Pfn2 ( Fig. 6d,e ). Because the N terminus of HDAC1 is a highly conserved catalytic domain and the C terminus contains a nuclear localization signal (NLS) [36] , profilin-2 likely interacted with the C terminus of HDAC1, which blocked the NLS and suppressed the nuclear localization of HDAC1. We also constructed C-HDAC1 (amino acids 1–322) and N-HDAC1 (amino acids 323–482) fragments ( Fig. 6b , lower panel) and examined the binding activities of profilin-2 with them. As shown in Fig. 6f , profilin-2 was able to interact with the full-length HDAC1 and C-HDAC1 fragments, but not the N-HDAC1 fragment. The above data indicate that the C terminus of profilin-2 and HDAC1 are important for their interaction, and the regulatory effect of profilin-2 on Smad expression is linked with its HDAC1-binding ability. 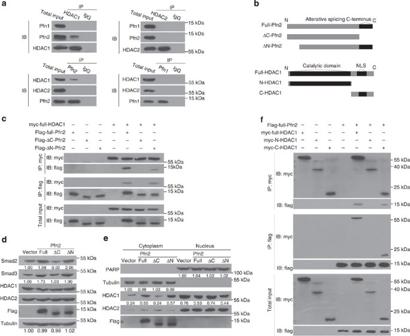Figure 6: The Pfn2–HDAC1 interaction is dependent on their C terminus. (a) Co-immunoprecipitation of Pfn1 and Pfn2 with HDAC1 and HDAC2. (b) Schematic illustration of full-length and deleted Pfn2 and HDAC1 proteins. NLS represent the nuclear localization signal. (c) The interaction between myc-tagged HDAC1 and flag-tagged Pfn2 fragment was detected by co-immunoprecipitation. (d) The expressions of Smads and HDACs were detected by western blotting. (e) The cellular localization of HDAC was detected by western blotting of the extracts of cytoplasmic and nuclear portions of cells. PARP was used as a marker of nucleus and tubulin was used as a marker of cytoplasm. (f) The interaction between flag-tagged Pfn2 and myc-tagged HDAC1 fragment was detected by co-immunoprecipitation. For all the western blotting results in this figure, one representative result of three experiments is shown. Figure 6: The Pfn2–HDAC1 interaction is dependent on their C terminus. ( a ) Co-immunoprecipitation of Pfn1 and Pfn2 with HDAC1 and HDAC2. ( b ) Schematic illustration of full-length and deleted Pfn2 and HDAC1 proteins. NLS represent the nuclear localization signal. ( c ) The interaction between myc-tagged HDAC1 and flag-tagged Pfn2 fragment was detected by co-immunoprecipitation. ( d ) The expressions of Smads and HDACs were detected by western blotting. ( e ) The cellular localization of HDAC was detected by western blotting of the extracts of cytoplasmic and nuclear portions of cells. PARP was used as a marker of nucleus and tubulin was used as a marker of cytoplasm. ( f ) The interaction between flag-tagged Pfn2 and myc-tagged HDAC1 fragment was detected by co-immunoprecipitation. For all the western blotting results in this figure, one representative result of three experiments is shown. Full size image HDAC1 is a target of Pfn2 in regulating the Smad expression To further confirm that profilin-2 regulates Smad2 and Smad3 expression by targeting HDAC1, we detected the binding intensity of HDAC1 to Smad promoter in profilin-2 overexpression or knockdown cells. Profilin-2 overexpression significantly decreased the binding of HDAC1 to Smad2 and Smad3 promoters, whereas its knockdown significantly increased the binding of HDAC1 to Smad2 and Smad3 promoters ( Fig. 7a,b ). Neither the overexpression nor knockdown of profilin-2 affected the binding of HDAC1 to Smad4 promoter ( Fig. 7c ). Knockdown of HDAC1 significantly rescued the Smad2 and Smad3 expression in profilin-2 knockdown cells, but had no effect on Smad4 expression ( Fig. 7d ). In addition, knockdown of HDAC1 reduced the suppressive effect of profilin-2 knockdown on soft agar colonies formation and matrigel invasion ability ( Fig. 7e,f ). Interestingly, due to the compensative increase of HDAC2 levels ( Fig. 7d ), knockdown of HDAC1 itself did not obviously increase the expression of Smad2 and Smad3, the soft agar colonies formation, and the invasion of A549 cells ( Fig. 7d–f ). These results are consistent with our previous observation that HDAC1 knockdown in AML12 cells led to a significant increase of HDAC2 level [37] . Further investigation showed that the knockdown of HDAC1 significantly increased the binding of HDAC2 to Smad2 and Smad3 promoters ( Fig. 7g,h ), but had no effect on the binding of HDAC2 to Smad4 promoters ( Fig. 7i ). The role of HDAC in the regulation of Smad2 and Smad3 expression was also verified by treating cells with Trichostatin A (TSA), a HDAC inhibitor. TSA treatment, in a time- and dose-dependent manner, upregulated the Smad2 and Smad3 expression and rescued the suppressive effect of profilin-2 knockdown on Smad expression ( Fig. 7j,k ). 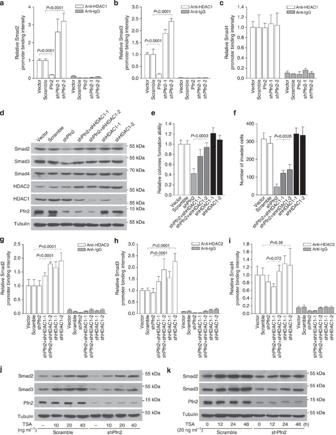Figure 7: The effect of HDAC1 on Smad expression. (a–c) The binding of HDAC1 to Smad promoter was detected by ChIP assay. Student’st-test is used for comparison of vector versus Pfn2 and ANOVA test for comparison of scramble, shPfn2-1 and shPfn2-2; all thePvalues are shown in the figure. Error bars represent the means±s.d. of three independent experiments. (d) Smad expression was detected by western blotting. One representative result of three experiments is shown. (e) The relative soft agar colony formation abilities were shown. ANOVA test;P=0.0003. Error bars represent the means±s.d. of four independent experiments. (f) The matrigel invasion ability was determined by the number of invaded cells. ANOVA test;P=0.0028. Error bars represent the means±s.d. of three independent experiments. (g–i) The binding of HDAC2 to Smad promoter was detected by ChIP assay. ANOVA test; all thePvalues are shown in the figure. Error bars represent the means±s.d. of three independent experiments. (j,k) The dose- and time-dependent effects of TSA on Smad expression. One representative result of three experiments is shown. ANOVA, analysis of variance. Figure 7: The effect of HDAC1 on Smad expression. ( a – c ) The binding of HDAC1 to Smad promoter was detected by ChIP assay. Student’s t -test is used for comparison of vector versus Pfn2 and ANOVA test for comparison of scramble, shPfn2-1 and shPfn2-2; all the P values are shown in the figure. Error bars represent the means±s.d. of three independent experiments. ( d ) Smad expression was detected by western blotting. One representative result of three experiments is shown. ( e ) The relative soft agar colony formation abilities were shown. ANOVA test; P =0.0003. Error bars represent the means±s.d. of four independent experiments. ( f ) The matrigel invasion ability was determined by the number of invaded cells. ANOVA test; P =0.0028. Error bars represent the means±s.d. of three independent experiments. ( g – i ) The binding of HDAC2 to Smad promoter was detected by ChIP assay. ANOVA test; all the P values are shown in the figure. Error bars represent the means±s.d. of three independent experiments. ( j , k ) The dose- and time-dependent effects of TSA on Smad expression. One representative result of three experiments is shown. ANOVA, analysis of variance. Full size image To briefly summarize our work, a schematic model is provided ( Fig. 8 ). In human lung cancer cells, profilin-2 binds HDAC1 and prevents its nuclear translocation to release its inhibitory effects on Smad2 and Smad3 transcription. High Smad2 and Smad3 levels render tumour cells more sensitive to TGF-β1, which increased VEGF and CTGF expression and TGF-β1-induced EMT, leading to the promotion of tumour growth and metastasis. Although profilin-1 has no obvious effect on lung cancer cell growth, it can negatively regulate the CTC concentration by inhibiting the invasion and/or intravasation of lung cancer cells. 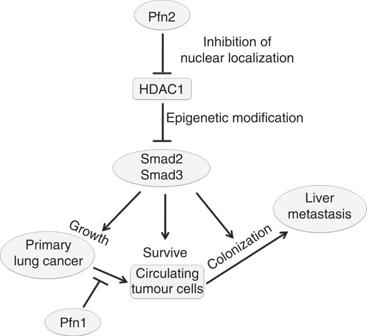Figure 8: Schematic illustration of the work. Pfn2 interacts with HDAC1 and suppresses the nuclear translocation of HDAC1, which epigenetically activated Smad2 and Smad3 expression, thereby promoting the growth of lung cancer cells and increasing the survival and liver colonization of CTC. Unlike Pfn2, Pfn1 functions as a suppressor of lung cancer invasion and intravasation, which can negatively impact the CTC level. Figure 8: Schematic illustration of the work. Pfn2 interacts with HDAC1 and suppresses the nuclear translocation of HDAC1, which epigenetically activated Smad2 and Smad3 expression, thereby promoting the growth of lung cancer cells and increasing the survival and liver colonization of CTC. Unlike Pfn2, Pfn1 functions as a suppressor of lung cancer invasion and intravasation, which can negatively impact the CTC level. Full size image Our current understanding of the mechanism underlying the alterations of Smad signalling during tumour progression is very limited. Although the mutations of type I and type II TGF-β receptors, Smad4 and Smad7 are common in different types of tumours, the mutations of Smad2 and Smad3 are rarely found [9] , [38] , [39] , implying that the alteration of Smad2 and Smad3 in tumour progression are not due to their genetic changes. In this study, we identified profilin-2 as a novel regulator of Smad2 and Smad3 by sequestering HDAC1 in cytoplasm to prevent its inhibitory effects. The findings not only broaden our understanding on the roles of profilin but also revealed an important molecular mechanism that controls TGF-β signalling in lung cancer cells. The previous studies on the regulation of TGF-β signalling are primarily focused on the genetic alterations and post-translational modifications (ubiquitination and sumoylation). The regulation at the epigenetic and transcription levels is not well understood. Thus, this investigation presented a novel insight into the regulatory mechanism of TGF-β signalling. At present, the therapeutic design targeting TGF-β signalling pathway in clinical trials for cancer treatment has been mostly focused on TGF-β antibodies, antisense oligonucleotides and receptor kinase inhibitors. Although the suppression of TGF-β signalling results in a significant reduction in tumour metastasis in mouse models, the clinical efficacy is not satisfactory. Because TGF-β signalling is involved in many normal physiological functions, these strategies can lead to unpredicted harmful side effects, generated by the long-term suppression of this pathway. In this study, we found that profilin-2 is a critical activator of TGF-β/Smad expression in human lung cancer cells. Profilin-2 is most abundantly expressed in brain and its expression in lung is very low [40] , it implies that profilin-2 is not an essential factor in the regulation of TGF-β/Smad signalling in normal lung tissues. Thus, the specific TGF-β signalling inhibitors that targeted profilin-2 will unlikely affect the TGF-β signalling in normal lung tissue, and may reduce the side effects of the general TGF-β signalling inhibitors. It is becoming clear that the effect of TGF-β on tumour initiation and progression is far more complex than previously assumed. For instance, the effects of TGF-β are known to be highly cell context dependent. The findings during the past decade that TGF-β is one of the most potent EMT inducer tremendously increased our understanding on the pathophysiological roles of TGF-β. Generally, the tumour suppressive effect of TGF-β depends on its ability to induce cell growth arrest and/or apoptosis. The tumour-promoting effect of TGF-β is highly related with its ability to induce EMT, angiogenesis and the anchorage-independent growth of cancer cells. TGF-β has very strong growth arrest and EMT induction effects in normal lung cells. Although the growth arrest effect of TGF-β has been largely abolished in lung cancers, TGF-β still can induce EMT, angiogenesis and anchorage-independent growth in many lung cancer cells. Due to the heterogeneity of the most cancers, the response or sensitivity of lung cancer cells to various signals including TGF-β can be different. The findings that profilin-2 strongly promotes xenograft growth and metastasis of A549 lung cancer cells and the low expression level of it in normal lung cells but significantly increased in lung cancer cells revealed that profilin-2–HDAC1 signalling can function as an important reprogramming factor in the progression of lung cancers, leading to the alterations in the expression profile of genes downstream of TGF-β. The high binding affinity with proline-rich motif is one of the most well characterized properties of profilin-2 molecules. Because a large number of proteins contain one or several proline-rich motifs, it’s likely that profilin-2 may be a regulator of various signalling pathways. For examples, profilin-2 may act as a modulator for PI3K-AKT signalling pathway, as AKT can phosphorylate several proline-rich substrates. The binding of profilin to actin monomer causes the enlongation of the uncapped actin filament and the disassembly of the capped actin filament, indicating that the binding of profilin to actin can result in different biological consequence. In summary, profilin-2 is not only a critical activator of the TGF-β signalling but also a potential regulator of the cell signalling network dynamics. It has been increasingly understood that critical steps during growth and metastatic progression of cancers involve increased angiogenesis, invasion and survival in the blood, and ability to colonize in metastatic sites. Profilin-1 knockdown increased the CTC concentration, but showed no effects on xenograft tumour growth. These results suggest that profilin-1 is an important suppressor for lung cancer cells invasion and intravasation. However, profilin-1 knockdown did not affect the distant metastasis of lung cancer cell. Because only a rare portion of invaded cells could survive in the peripheral blood and surviving CTC successfully form distant metastasis are even rarer [41] , [42] , the invasion of cancer cells does not necessarily ensure their distal metastatic growth. Unlike profilin-1, the increased CTC concentration caused by profilin-2 overexpression was accompanied by a significantly increased tumour size. Profilin-2 also significantly enhances the survival rate and liver colonization ability of CTC. Thus, it is possible that profilin-1 and profilin-2 are important for the progression of lung cancer at different stages. Profilin-1 increases the ability of lung cancer cells to escape from the primary tumour, while profilin-2 increases the survival and outgrowth of cancer cells. Knockdown of profilin-1 increased the lung cancer invasion, which is consistent with the previously reported effect of profilin-1 in breast cancer [20] , [21] , [23] . Mouneimne et al. [24] recently reported that profilin-1 promotes, but profilin-2 suppresses, the migration and invasion of breast cancer cells. The discrepancy between their results and our findings may be partially be due to the differences of tissue and cell systems used, since the potential roles of profilin in human cancer are highly dependent on cell context and environment. Although profilin-1 has no effect on the lung metastasis formation and its overexpression cannot rescue the profilin-2 knockdown-mediated suppression of lung and liver metastasis, both its overexpression and knockdown can decrease the liver metastasis mediated by profilin-2 overexpression (data not shown). These results indicate that profilin-2 plays an important role in lung and liver metastasis, and a quantitative relationship between profilin-2 and profilin-1 has been implicated in their functions. HDAC1 has a NLS sequence and is primarily located in the nucleus. We found that profilin-2 can sequestrate HDAC1 in the cytoplasm, which increased the transcription of Smad and thus promoted lung cancer progression. These findings broadened our understanding on the molecular mechanism of HDAC1 function. Moreover, we found that the HDAC2 expression is significantly upregulated in the HDAC1 knockdown cells. HDAC2 compensated the HDAC1 loss to repress the Smad2 and Smad3 expression. Although profilin-2 overexpression significantly suppressed the nuclear localization of HDAC1, the expression of HDAC2 was not affected by profilin-2 overexpression. These results imply that the compensative effect of HDAC2 is triggered by downregulated HDAC1 expression, but not by the decreased nuclear location of HDAC1. Alteration of epigenetic regulation of gene expression has been implicated in tumour development and progression. HDACs play a central role in the epigenetic regulation of genes expression. HDACs have become attractive anticancer targets because HDAC inhibitors can induce tumour cell apoptosis, growth arrest, senescence, differentiation and immunogenicity, and inhibit angiogenesis in many cases. The most successful clinical application of HDAC inhibitors is the use of vorinostat and romidepsin against refractory cutaneous and peripheral T-cell lymphoma. Currently, the efficacy of >20 different HDAC inhibitors tested in the clinic has been largely restricted to haematological malignancies. Whereas the effect of HDAC inhibitors used in the treatment of solid tumours are disappointing [43] , [44] , it has also been shown that HDAC inhibitors can induce EMT in prostate cancer cells [45] . HDAC1 and HDAC2 have been reportedly shown to function as tumour suppressors in epidermis and lymphomas [46] , [47] , [48] . In this study, we also showed that HDAC1 is a negative regulator of Smad2 and Smad3. TSA treatment can increase the expression of Smad2 and Smad3, suggesting that HDAC1 is a potent suppressor of lung cancer progression. Thus, cautions should be exercised when using HDAC inhibitor as anticancer drugs. Cell culture All the cells used in this study were purchased originally from American Type Culture Collection. 293T and A549 cells were grown in Dulbecco’s modified Eagle’s medium containing 10% fetal bovine serum (FBS) supplemented with penicillin (100 U ml −1 ) and streptomycin (100 mg ml −1 ). H1650, HCC827, H358, H446 and H1299 cells were grown in 1,640 medium containing 10% FBS supplemented with penicillin (100 U ml −1 ) and streptomycin (100 mg ml −1 ). Primary hepatocytes isolated from C57BL/6 mice were grown in a 1:1 mixture of Dulbecco’s modified Eagle’s medium and Ham’s F12 medium containing 10% FBS and supplemented with insulin–transferrin–selenium-X, dexamethasone (40 ng ml −1 ), penicillin (100 U ml −1 ) and streptomycin (100 mg ml −1 ). The cells were incubated at 37 °C in a humidified atmosphere of 5% CO 2 . Antibodies and reagents TGF-β1 was purchased from Chemicon (Millipore, Billerica, MA, USA). Beta-tubulin (ab21057, 1:2,000 for western blotting assay) and profilin-2 (ab55611, 1:2,000 for western blotting) antibodies were purchased from Abcam (Cambridge, UK). Antibodies against Smad2 (3103, 1:500 for western blotting, 1:100 for immunohistochemistry staining), Smad3 (9513S, 1:500 for western blotting, 1:100 for immunohistochemistry staining), profilin-1 (3237, 1:1,000 for western blotting), acetyl-histone H2BK12 (#2575, 1:50 for chromatin immunoprecipitation (ChIP) assay), acetyl-histone H2AK5 (#2576, 1:50 for ChIP assay), tri-methyl-histone H3K4 (#9751S, 1:50 for ChIP assay), tri-methyl-histone H3K9 (#9754S, 1:50 for ChIP) and tri-methyl-histone H3K27 (9756S, 1:50 for ChIP assay) were from Cell Signaling Technology (Boston, MA, USA). Flag antibody (F3165.2MG, 1:1,000 for western blotting, 1:50 for ChIP assay) was obtained from Sigma (St Louis, MO, USA). Antibody for acetyl-histone H3K9/14 (06–599B, 1:50 for ChIP assay) was purchased from Upstate Biotechnology (Lake Placid, NY, USA). Cell invasion assays The cell invasion assays were performed using trans-well migration chambers (8 μm pore size; Costar) according to the vendor’s instructions. Briefly, the insert of the wells were first coated with 40 μl of BD matrigel and then 20,000 cells were plated into the insert of the well. After cultured at 37 °C in a humidified atmosphere of 5% CO 2 for 24 h, the invaded cells were calculated under microscopy. Preparation of cell lysates and western blotting Cells were lysed in 10 mM Tris (pH 7.4), 1 mM EDTA, 0.5 mM EGTA, 150 mM NaCl, 1% Triton X-100, 50 mM NaF, 10 mM Na 4 P 2 O 7 ·10 H 2 O, 5 μg ml −1 aprotinin, 5 μg ml −1 leupeptin and 1 mM PMSF. Western blot analysis was performed as previously described [49] . Protein samples were electrophoresed on SDS–polyacrylamide gels and transferred to nitrocellulose membranes. The membranes were blocked with 5% skim milk in Tris-buffered saline containing 0.1% Tween-20 (TBST) and subsequently incubated with primary antibody overnight at 4 °C. The membranes were washed again with TBST for three times at room temperature and then incubated with a horseradish peroxidase-conjugated secondary antibody for 1 h, followed by a 5-min wash three times. Protein bands were visualized with the Super Signal Reagents (Pierce, Thermo Fisher Scientific, Rockford, IL, USA). Extended scans of immunoblots are shown in Supplementary Figs 10–13 . Real-time PCR Real-time PCR was performed using Power SYBR Green PCR Master Mix with Applied Biosystems 7500 Fast Real-Time PCR systemaccording to the vendor’s instructions. In brief, incubation cycles were as follows: 95 °C for 10 min, 95 °C for 15 s and 60 °C for 1 min. Amplification was completed by 40 cycles and the melting curves were measured. The sequences of primers used for Real-time PCR assay are listed in Supplementary Table 2 . 3 H-thymidine incorporation analysis The assay was conducted as previously described [50] . Cells were grown in 35-mm dishes to about 80% confluence, and were labelled with 3 H-thymidine (0.1 μCi ml −1 ) in the last 4 h of incubation. The medium was discarded and the cells were washed with ice-cold PBS three times, followed by adding 500 μl of 12% trichloro acetic acid. The dishes were maintained on ice for 30 min and washed again with PBS three times. The acid-insoluble material was redissolved in 300 μl lysis buffer (1% SDS, 0.2 N NaOH) and moved into scintillation vials, mixed with 2.5 volumes of Biodegradable Counting Scintillant. The DNA-associated [ 3 H]-radioactivity was determined by liquid-scintillation spectrometry (Wallac 1409, Pharmacia). Immunofluorescent staining and confocal microscopy Cells were grown on glass slides for 2 days, then washed quickly with PBS and fixed in 4% Paraformaldehyde (PFA) for 15 min. The samples were subjected to probing with the appropriate primary and secondary antibodies. F-actins were stained with phalloidin (Invitrogen, A22281) and the nuclei were stained with 4′,6′-diamidino-2-phenylindole (Invitrogen, P-36931) according to the vendor’s instructions. The fluorescence was visualized under confocal microscopy (Leica TCS SP5 MP). Immunoprecipitation assay Cells were lysed in ice-cold RIPA buffer (phosphate-buffered solution containing 1% Nonidet P-40, 0.1% SDS and 0.5% sodium deoxycholate) supplemented with 50 mM NaF, 1 mM Na 3 VO 4 , 10 mM Na 4 P 2 O 7 , 5 μg ml −1 aprotinin, 5 μg ml −1 leupeptin and 1 mM PMSF. After the insoluble fraction was removed by centrifugation at 4 °C for 10 min at 12,000 r.p.m., the whole-cell lysates were pre-cleared using protein-A/G sepharose. Immunoprecipitation was performed by incubating the above lysates with protein-G sepharose that was pre-absorbed with 2 μg of the indicated primary antibodies at 4 °C overnight, using an equal amount of normal IgG as negative control. After extensive washing, the sepharose beads were boiled in 50 μl of 1 × SDS–polyacrylamide gel electrophoresis loading buffer for 5 min at 95 °C. The eluted proteins were then subjected to western blotting. ChIP assay and detection of histone acetylation/methylation The ChIP assay was performed using the EZ-Zyme Chromatin Prep Kit (Millipore, Billerica, MA, USA) according to the manufacture’s protocol. Briefly, Cells were fixed with 1% formaldehyde and incubated at room temperature for 10 min. Then 10 × glycine was added to dishes and incubated for 5 min. Ez-Zyme enzymatic cocktail was used to cleave the DNA. Protein–DNA complexes were immunoprecipitated with specific antibodies. The DNA–protein immunocomplexes were collected with protein-A/G agarose beads, washed and eluted with freshly prepared elution buffer (1% SDS, 0.1 M NaHCO 3 ). The mixture was further incubated with 5 M sodium chloride at 65 °C for 4 h to reverse crosslinked DNA–protein complexes. Protein K (10 mg ml −1 ) was added to the samples and incubated for 1 h at 45 °C. DNA samples were then purified with phenol/chloroform, precipitated with ethanol, and resuspended in TE buffer. Real-time PCR reaction was performed to quantify target DNA fragment. Antibodies for acetyl-histone H2BK12, H2AK5 and H3K9/14 were used in the ChIP assay to detect the acetyl-histone levels of Smad promoters. Antibodies for tri-methyl-histone H3K4, H3K9 and H3K27 were used for ChIP assay to detect the methyl-histone levels of Smad promoters. HDAC1 and HDAC2 antibodies were used for ChIP assay to detect the binding intensity of HDAC to Smad promoter. Three sets of primers that cover Smad promoters from about −2 kb to 0 b were used for ChIP assay. The primer sequences were shown in the Supplementary Table 2 . The results were shown as the relative average ChIP intensities of the three sets primers. Detection of CTCs The blood from mice was isolated and red blood cells were lysed. The total RNA was extracted using Trizol reagent. Then, mRNA was reverse transcribed at 42 °C for 30 min using ReverTra Ace-α (Toyobo). The relative CTCs were determined as a ratio of human tubulin expression (detected by a set of human specific primers: forward, 5′-CAGATGCCCAGTGACAAGACC-3′ and reverse, 5′-CAATGACCGTAGGCTCCAGAT-3′) to mouse GAPDH expression (detected by a set of mouse specific primers: forward, 5′-AGGTCGGTGTGAACGGATTTG and reverse, 5′-GGCCTCACCCCATTTGATGT-3′). Animal experiments and ethical approval The lung cancer tissue chips (HLug-Ade150sur-01, OD-CT-Rslug03-002) were purchased from Shanghai Superchip Company. Informed consent was not required, as we used archival samples from Shanghai National Engineering Research Center for biological chip that remained anonymous. Female athymic nude mice (BALB/cASlac-nu) were purchased from Shanghai SLAC Laboratory Animal Center. All animals received standard care, and study protocols were approved by the Shanghai Experimental Animal Center of Chinese Academy of Sciences (Approval Number: IBCB-SPF0041). Animals were maintained in individually ventilate cages (no more than five mice per cage) in a specific pathogen-free animal facility with a climate-controlled environment on a 12-h light/12-h dark cycle and fed ad libitum with regular rodent chow. Seven- to 9-week-old female mice were used for xenograft tumour growth and metastasis assay. For xenograft tumour growth assay, 10,000,000 cells were subcutaneously injected per mouse. The mice injected with profilin-2-overexpressing and knockdown A549 cells were euthanized by CO 2 overdose 6 weeks after injection. Tumour sizes were measured once per week. The tumour volume was calculated as V =3.14 × D average diameter 3 /6. The maximally allowed volume for individual tumours was 6,000 mm 3 and the tumours were isolated and weighed after mice were euthanized. For tumour metastasis assay, 1,000,000 cells were used for tail-vein injection per mouse. Animals were euthanized and tissues were harvested 2 months after injection. Blood for analysis was collected from retro-orbital sinus under isoflurane anaesthesia. Animals were euthanized when one of the following signs of morbidity were observed: individual tumour volume >6,000 mm 3 , significant tumour ulceration (>1 cm), significant weight loss (>20%), severe injure that induce secondary infection and dehydration, and inability to move, feed, groom and defecate. Qualified animal feeders and researchers observed animals daily, and consensus decision was made for each mouse. The raw data underlying the tumour growth curves shown in Figs 2b and 4b and Supplementary Fig. 2d are provided as Supplementary Data 1–3 . Immunohistochemistry staining assay Experiments were performed according to the protocols provided by the Cell Technology Platform of SIBCB ( http://www.sibcb.ac.cn/cp13-4.asp ) with minor modifications. In brief, the paraffin sections were deparaffinized in xylene, hydrated in decreasing concentrations of ethanol, retrieved in an antigen retrieval buffer and treated with 3% H 2 O 2 . Then, the sections were blocked with 3% BSA, and followed by incubating with specific primary antibody and horseradish peroxidase-conjugated secondary antibody. The bound antibody was revealed by 3,3'-diaminobenzidine (DAB)/H 2 O 2 substrate and the nucleus was stained with haematoxylin. Preparation of mouse primary hepatocytes Six-week-old female C57BL/6 mice (C57BL/6Slac) were purchased from the Shanghai Experimental Animal Center of Chinese Academy of Sciences. Primary mouse hepatocytes were isolated by two-step in situ collagenase perfusion procedures as described previously [51] . Briefly, livers were perfused in situ through the portal vein with calcium- and magnesium-free Earle’s Basic Salt Solution (EBSS) for 3 min at a rate of 5 ml min −1 , followed by EBSS for another 3 min at 5 ml min −1 . Then, the liver was digested using 0.5 mg ml −1 of type IV collagenase in EBSS for 10 min at 37 °C. The hepatocytes were collected by centrifugation and seeded in Dulbecco’s modified Eagle’s medium containing 10% FBS, and media was changed 6 h after incubation. Cultures were maintained at 37 °C in a humidified atmosphere of 5% CO 2 in Dulbecco’s modified Eagle’s medium with 10% FBS, 100 units per millilitre penicillin and 100 g ml −1 streptomycin. Flow cytometry analysis Propidium iodide (Invitrogen, P3566) staining was used to detect the cell cycles. Briefly, cells in 35-mm dishes were trypsinized and fixed with 70% ethanol for >1 h. Cells were pelleted and washed with PBS plus 20 mM EDTA. After being incubated with RNase (1 mg ml −1 ) at 37 °C for 1 h, cells were stained with propidium iodide (30 mg ml −1 ) and DNA content was analysed using BD FACS Calibur. Luciferase assay The Smad promoters that range from about −2 kb to +200 b were cloned into the pGL3-Basic vector. The primers used for Smad2 promoter construction are: 5′-CCCTAGTGGCTCTGGAAAGAGGA-3′ (forward) and 5′-AGCGGAGGAGGAAAGGAACGA-3′ (reverse). The primers used for Smad3 promoter construction are: 5′-GCTGGGTGCAGTCTCAAGATCG-3′ (forward) and 5′-CTCCCACGGCGAAGAGAAGAG-3′ (reverse). The luciferase activities (firefly luciferase and Renilla luciferase) were determined using the Dual-Luciferase Reporter Assay System (E1910, Promega). In all reporter assays, the Renilla luciferase activity was measured to correct for transfection efficiency. H-score quantification The H-score method assigned a score of 0–9 to each sample, based on the percentage of cells stained at different intensities viewed under the microscope. The discriminatory threshold was set at 5, samples with H-score ≥5 were classed as high profilin-2 (or Smad3) expression, while samples with H-score <5 were classed as low profilin-2 (Smad3) expression. Statistical analysis Quantitative data are expressed as the means±s.e.m. or s.d. Statistical significance was determined by Student’s t -test for comparison of two groups and analysis of variance with post hoc tests for more than groups. A P value of <0.05 was considered statistically significant. How to cite this article: Tang, Y.-N. et al. Epigenetic regulation of Smad2 and Smad3 by profilin-2 promotes lung cancer growth and metastasis. Nat. Commun. 6:8230 doi: 10.1038/ncomms9230 (2015).